Insights into bird wing evolution and digit specification from polarizing region fate maps The proposal that birds descended from theropod dinosaurs with digits 2, 3 and 4 was recently given support by short-term fate maps, suggesting that the chick wing polarizing region—a group that Sonic hedgehog -expressing cells—gives rise to digit 4. Here we show using long-term fate maps that Green fluorescent protein -expressing chick wing polarizing region grafts contribute only to soft tissues along the posterior margin of digit 4, supporting fossil data that birds descended from theropods that had digits 1, 2 and 3. In contrast, digit IV of the chick leg with four digits (I–IV) arises from the polarizing region. To determine how digit identity is specified over time, we inhibited Sonic hedgehog signalling. Fate maps show that polarizing region and adjacent cells are specified in parallel through a series of anterior to posterior digit fates—a process of digit specification that we suggest is involved in patterning all vertebrate limbs with more than three digits. Bird wing digits anatomically resemble digits 1, 2 and 3 of the hands of basal Triassic theropod dinosaurs such as Herrerasaurus and Eodromaeus , and the fossil record shows a progressive loss of digits 4 and 5 in the tetanuran theropod lineage that gave rise to modern birds [1] , [2] , [3] , [4] , [5] ( Fig. 1a ). However, it has been suggested that bird wing digits arise in the embryo in digit positions 2, 3 and 4 because all vertebrate limbs are thought to have a 'primary axis' of cartilage condensation running through cells that give rise to digit 4 (ref. 6 ; Fig. 1b , red line). In addition, transient digit condensations have been reported in putative digit 1 and 5 positions [6] , although it is debated whether the digit 1 condensation is a true digit primordium, and an additional posterior condensation has also been detected [7] . Genetic fate maps of polarizing region cells expressing LacZ under the Shh promoter in the mouse limb, which has five digits (1 to 5), demonstrated that the digit 4 position is within the polarizing region—a small population of Sonic hedgehog ( Shh )-expressing cells at the posterior margin of vertebrate limb buds—and that digits 4 and 5 arise entirely from polarizing region cells [8] ( Fig. 1b,c ). Recently, short-term dye-based fate maps also suggest that the digit 4 position is in polarizing region of both the chick wing bud ( Fig. 1d,e ) and the chick leg bud with four digits (I–IV), and that all of digit 4 comes from the polarizing region [9] . This supports the so-called 'frame-shift' or 'identity-shift', which proposes that during the evolution of the theropod hand/bird wing, digits with the anatomies of ancestral digits 1, 2 and 3 developed in ancestral positions 2, 3 and 4 (ref. 10 ) and theropods lost digits 1 and 5 (ref. 9 ) ( Fig. 1d,e ). This pattern of digit loss is only indicated in the derived Jurassic theropod Limusaurus [11] of the ceratosaurian lineage of theropods that did not give rise to modern birds ( Fig. 1a ). 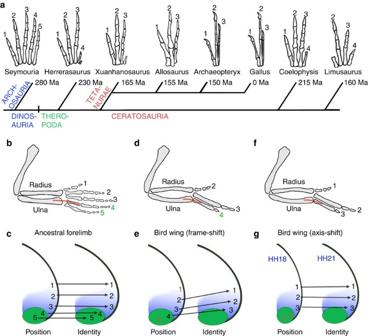Figure 1: Evolution of bird wing digits from dinosaur hand digits. (a) Fossil record indicates birds evolved from the tetanuran lineage of basal theropod dinosaurs that progressively lost digits 4 and 5 in the hand (adapted from Weishampelet al.3). (b,c) Proposed conserved primary axis of cartilage condensation for ancestral limbs (red line,b) and digits 4 and 5 (green oval,c) derived from the polarizing region as in mouse limbs. (d,e) Frame-shift hypothesis predicts birds evolved from theropods with a 2, 3 and 4-digit pattern. Primary axis in digit 4 position (red line,d)—digits 1 and 5 lost (red numbers), polarizing region cells give rise to a digit that is specified with a digit 3 identity in the bird wing (e). (f,g) Data presented in this study are consistent with axis-shift hypothesis, in which birds evolved from theropods with a 1, 2 and 3-digit pattern. Primary axis in digit 3 position (red line,f)—digits 4 and 5 lost (red numbers), polarizing region cells do not give rise to a digit 4 in the bird wing and digits 1, 2 and 3 specified in ancestral positions between Hamburger and Hamilton (HH) stages 18 and 21 (g). Note Gallus is the chicken. Figure 1: Evolution of bird wing digits from dinosaur hand digits. ( a ) Fossil record indicates birds evolved from the tetanuran lineage of basal theropod dinosaurs that progressively lost digits 4 and 5 in the hand (adapted from Weishampel et al . [3] ). ( b , c ) Proposed conserved primary axis of cartilage condensation for ancestral limbs (red line, b ) and digits 4 and 5 (green oval, c ) derived from the polarizing region as in mouse limbs. ( d , e ) Frame-shift hypothesis predicts birds evolved from theropods with a 2, 3 and 4-digit pattern. Primary axis in digit 4 position (red line, d )—digits 1 and 5 lost (red numbers), polarizing region cells give rise to a digit that is specified with a digit 3 identity in the bird wing ( e ). ( f , g ) Data presented in this study are consistent with axis-shift hypothesis, in which birds evolved from theropods with a 1, 2 and 3-digit pattern. Primary axis in digit 3 position (red line, f )—digits 4 and 5 lost (red numbers), polarizing region cells do not give rise to a digit 4 in the bird wing and digits 1, 2 and 3 specified in ancestral positions between Hamburger and Hamilton (HH) stages 18 and 21 ( g ). Note Gallus is the chicken. Full size image Short-term dye-labelling techniques have limitations, as they do not show which tissues labelled cells give rise to. Therefore, to understand how digit patterns are generated, we made polarizing region grafts from transgenic Green fluorescent protein ( Gfp )-expressing chicken embryos [12] into limb buds of normal embryos to make long-term fate maps. Here we show that the chick wing polarizing region does not give rise to a digit supporting the proposal that the digits of the bird wing are 1, 2 and 3 having evolved from theropod dinosaurs that had the same digits ( Fig. 1f,g ). Additionally, we reveal that chick leg polarizing region cells give rise to the most-posterior digit and are promoted through a series of anterior to posterior digit fates, leading to a new model of how limbs with more than three digits are generated. The chick wing polarizing region gives rise to the posterior margin of digit 4 To make long-term fate maps, we replaced chick wing polarizing regions with Gfp -expressing polarizing regions. When replaced at stages 18 (onset of Shh transcription), 19 and 20, the polarizing region gave rise to a narrow band of cells extending along the entire posterior margin of digit 4 in day 10 wings ( Fig. 2a ). To check that we are only transplanting polarizing region cells, we replaced chick wing polarizing regions at stage 19 and analysed Shh expression immediately in the donor embryo and 4 h later in the host embryo. This showed that Shh transcripts could not be detected in the donor bud and were present only in the graft in the host bud ( Fig. 2b ). When the dorsal surface of the wing is viewed in ovo at stage 30 (day 7), GFP-expressing cells seem to contribute to the cartilage condensation of digit 4 ( Fig. 2c ) and are superficially similar to whole-mounts of dye-labelled polarizing region fate maps [9] , [13] , [14] . But longitudinal ( Fig. 2d —plane shown in Fig. 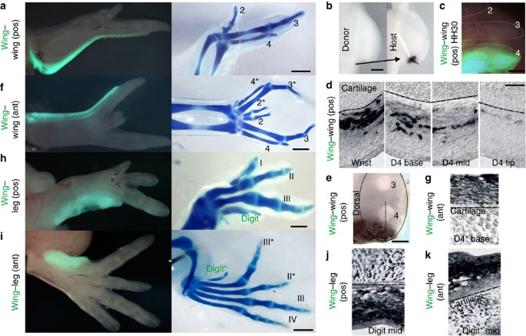Figure 2: Chick wing polarizing region fate maps. (a)Gfp-expressing polarizing regions grafted in place of host (pos, posterior) polarizing regions contribute to the posterior margin of digit 4 (n=11/14). (b)Shhexpression in donor wing bud 0 h and host wing bud 4 h after polarizing region replaced (n=3/3). (c) Cells derived from polarizing region seem to co-localize with digit 4 cartilage condensation in day 7 whole mounts (n=2/2). (d,e) Longitudinal (d,n=2/2, plane shown by dashed line ine) and transverse (e,n=2/2) sectionin situsshowingGfpexpression in soft tissue adjacent to day 10 digit 4 cartilage. (f)Gfp-expressing polarizing regions grafted to anterior (ant) margins contribute to the posterior margin of duplicate (*) chick wing digit 4 (n=21/21). (g) Longitudinal sectionin situshowingGfpexpression in soft tissue adjacent to duplicate (*) day 10 digit 4 cartilage (n=3/3). (h,i)Gfp-expressing chick wing polarizing regions grafted in place of a chick leg polarizing region (h) and to the anterior margin of a chick leg bud (i) give rise to digits (n=7/10). (j,k) Longitudinal sectionin situshowingGfpexpression in soft tissue and cartilage of digit derived from chick wing polarizing region grafted to the posterior (j) or anterior (k) margin of a chick leg bud (n=2/2). Scale bars:a,f,I—1 mm;b,c—100 μm; d—50 μm (g,j,k—same scale);e—150 μm;h—750 μm. 2e ) and transverse ( Fig 2e ) sections show that Gfp -expressing cells are restricted to the posterior margin of the handplate in soft tissues adjacent to, but not in the digit 4 cartilage rudiment. Detailed examination of Gfp expression in longitudinal sections through the centre of digit 4 revealed a progressive reduction in Gfp -positive cells in the soft tissue of digit 4 going from proximal to distal ( Fig. 2d ). We also initiated a duplicate digit pattern by grafting Gfp -expressing polarizing regions to the anterior margins of stage 19/20 host chick wing buds [15] , [16] . Again, the wing polarizing region gave rise to a narrow band of soft tissue adjacent to the cartilage rudiment of the duplicate digit 4 in patterns such as 4–3–2–2–3–4 ( Fig. 2f,g ). Figure 2: Chick wing polarizing region fate maps. ( a ) Gfp -expressing polarizing regions grafted in place of host (pos, posterior) polarizing regions contribute to the posterior margin of digit 4 ( n =11/14). ( b ) Shh expression in donor wing bud 0 h and host wing bud 4 h after polarizing region replaced ( n =3/3). ( c ) Cells derived from polarizing region seem to co-localize with digit 4 cartilage condensation in day 7 whole mounts ( n =2/2). ( d , e ) Longitudinal ( d , n =2/2, plane shown by dashed line in e ) and transverse ( e , n =2/2) section in situs showing Gfp expression in soft tissue adjacent to day 10 digit 4 cartilage. ( f ) Gfp -expressing polarizing regions grafted to anterior (ant) margins contribute to the posterior margin of duplicate (*) chick wing digit 4 ( n =21/21). ( g ) Longitudinal section in situ showing Gfp expression in soft tissue adjacent to duplicate (*) day 10 digit 4 cartilage ( n =3/3). ( h , i) Gfp -expressing chick wing polarizing regions grafted in place of a chick leg polarizing region ( h ) and to the anterior margin of a chick leg bud ( i ) give rise to digits ( n =7/10). ( j , k ) Longitudinal section in situ showing Gfp expression in soft tissue and cartilage of digit derived from chick wing polarizing region grafted to the posterior ( j ) or anterior ( k ) margin of a chick leg bud ( n =2/2). Scale bars: a , f , I —1 mm; b , c —100 μm; d—50 μm ( g , j , k —same scale); e —150 μm; h —750 μm. Full size image Previous experiments showed that a wing digit is produced when a stage 20 chick wing polarizing region is grafted to the anterior margin of a chick leg bud [17] , although not when a stage 22 quail wing polarizing region was grafted [9] . We confirmed by grafting stage 19/20 Gfp -expressing chick wing polarizing regions, either to the anterior margin of chick leg buds or in place of the endogenous leg polarizing region, that, under these circumstances, the wing polarizing region can give rise to a digit in day 10 legs ( Fig. 2 h,i ). Examination of Gfp expression in longitudinal sections through the centre of these digits revealed that both soft tissues and cartilage were derived from the wing polarizing region ( Fig. 2j,k ). Timing of chick wing digit specification by Shh signalling To determine when cells in the chick wing bud are specified with digit identities, we replaced stage 18/19 wing polarizing regions with Gfp -expressing polarizing regions and then inhibited Shh signalling by adding cyclopamine at a series of later time points. Consistent with previous reports [14] , [18] , cyclopamine application at stage 18/19 ( ∼ 4 h after the onset of Shh transcription) resulted in wings with a single digit 2 pattern ( Fig. 3a ); at stage 19/20 ( ∼ 8 h of Shh transcription), a 2–3 pattern ( Fig. 3b ) and at stage 21( ∼ 12 h of Shh transcription), a 2–3–4 pattern as in normal wings ( Fig. 2a ). In all these different patterns, the polarizing region gave rise to a thin line of cells just along the posterior margin of the handplate of day 10 wings and did not form a digit ( Fig. 3a–c ), as in normal wings ( Fig. 2a ). We also replaced wing bud polarizing regions with Gfp -expressing polarizing regions and inhibited expansion of the wing bud by application of trichostatin A (TSA) at stage 19 (ref. 14 ). We still found that the polarizing region gave rise to thin stripe of cells along the posterior margin of day 10 wings that had a digit 3–4 pattern ( Fig. 3d ) or a single digit 4 ( Fig. 3e,f ). To some TSA-treated wing buds, we then added cyclopamine after 24 h (single-headed arrow, Fig. 3f ) to shorten the duration of Shh signalling in the unexpanded digit-forming field, resulting in wings with a single digit 3 ( Fig. 3 g ). Again, the polarizing region did not give rise to a digit, but instead gave a thin line of cells along the posterior margin of the wing ( Fig. 3g ). These data show that the wing bud polarizing region never gives rise to a digit in the wing, but always extends along the posterior margin during outgrowth. 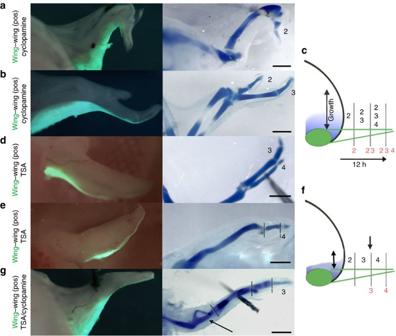Figure 3: Timing of chick wing digit specification. (a–c) Inhibition of Shh signalling in the wing bud using cyclopamine at stage 18/19 results in a single digit 2 pattern (a,n=3/8 and red number,c) and at stage 19/20, a 2–3 digit pattern (b,n=4/5 and red numbers,c)—Gfp-expressing wing polarizing region cells do not contribute to digit skeletons and extend along the posterior margin to the distal tip of the adjacent digit (a–c). (c) Digit progenitors adjacent to the polarizing region (green oval) are transiently specified and promoted through a series of anterior identities (black numbers) by a gradient of paracrine Shh signalling (blue) over 12 h; Shh-dependent growth (black double-headed arrow) allows entire digit-forming field adjacent to polarizing region to progressively give rise to one digit, two digits and then three digits; the polarizing region cell lineage tapers during outgrowth (green lines,c). (d–g) TSA application reduces expansion of digit-forming field (indicated by shortened double-headed arrow) and anterior digits are lost giving digits 3–4 (d,n=2/3) and digit 4 patterns (e,f,n=7/8, phalanges shown by dashed lines). Application of cyclopamine (single-headed black,f) after TSA prevents posterior specification and a digit 3 forms (g,n=11/14, reduced forearm shown by arrow and phalanges by dashed lines). In all casesGfp-expressing polarizing regions do not contribute to digit skeleton development,d–g). Scale bars:a—500 μm;b—750 μm;d—500 μm;e,f—250 μm. Figure 3: Timing of chick wing digit specification. ( a – c ) Inhibition of Shh signalling in the wing bud using cyclopamine at stage 18/19 results in a single digit 2 pattern ( a , n =3/8 and red number, c ) and at stage 19/20, a 2–3 digit pattern ( b , n =4/5 and red numbers, c )— Gfp -expressing wing polarizing region cells do not contribute to digit skeletons and extend along the posterior margin to the distal tip of the adjacent digit ( a – c ). ( c ) Digit progenitors adjacent to the polarizing region (green oval) are transiently specified and promoted through a series of anterior identities (black numbers) by a gradient of paracrine Shh signalling (blue) over 12 h; Shh-dependent growth (black double-headed arrow) allows entire digit-forming field adjacent to polarizing region to progressively give rise to one digit, two digits and then three digits; the polarizing region cell lineage tapers during outgrowth (green lines, c ). ( d – g ) TSA application reduces expansion of digit-forming field (indicated by shortened double-headed arrow) and anterior digits are lost giving digits 3–4 ( d , n =2/3) and digit 4 patterns ( e , f , n =7/8, phalanges shown by dashed lines). Application of cyclopamine (single-headed black, f ) after TSA prevents posterior specification and a digit 3 forms ( g , n =11/14, reduced forearm shown by arrow and phalanges by dashed lines). In all cases Gfp -expressing polarizing regions do not contribute to digit skeleton development, d – g ). Scale bars: a —500 μm; b —750 μm; d —500 μm; e , f —250 μm. Full size image The chick leg polarizing region gives rise to digit IV To gain insights into how a more complex digit pattern than that of the chick wing is specified, we replaced chick leg polarizing regions with Gfp -expressing polarizing regions. When replaced at stage 19 and stage 20, the chick leg polarizing region gave rise to digit IV in day 10 embryos ( Fig. 4a ). For detailed cellular analysis, we replaced the host leg polarizing region with a Gfp -expressing polarizing region graft at stage 20 and examined expression of Gfp in day 10 embryos in longitudinal sections. This revealed that Gfp -expressing cells were found throughout the soft tissue and cartilage skeleton of digit IV, but not of digit III ( Fig. 4b ). To extend this analysis, we initiated a duplicate digit pattern [17] by grafting Gfp -expressing polarizing regions to the anterior margin of stage 19/20 leg buds. Again, the leg polarizing region gave rise to the entire duplicate digit IV in patterns such as IV–III–II–III–IV ( Fig. 4c ). Expression of Gfp could be observed throughout the cartilage skeleton and soft tissues in longitudinal sections of the duplicate digit IV, but not digit III ( Fig. 4d ). 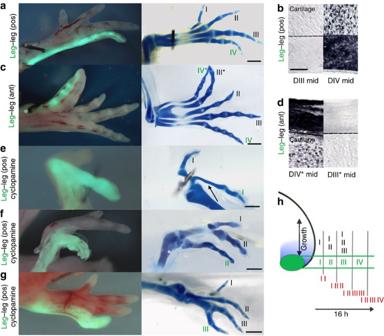Figure 4: Chick leg polarizing region fate maps and timing of digit specification. (a)Gfp-expressing polarizing regions grafted in place of host (pos, posterior) polarizing regions give rise to digit IV (n=7/9). (b) Longitudinal sectionin situshowingGfpexpression in soft tissue and cartilage of digit IV, but not digit III (n=2/2). (c)Gfp-expressing polarizing regions grafted to anterior (ant) margins give rise to duplicate (*) chick wing digit IV (n=9/9). (d) Longitudinal sectionin situshowingGfpexpression in soft tissue and cartilage of duplicate (*) digit IV, but not duplicate digit III (n=1/1). (e–g) Inhibition of Shh signalling in the leg bud using cyclopamine at stage 18/19 results in a I–I digit pattern (e,n=2/2 and red numbers,h), at stage 19/20, a I–II–II pattern (f,n=4/4 and red numbers,h) and at stage 21, a I–II–III–III pattern (g,n=6/7 and red numbers,h), leg polarizing region cells always give rise to the most-posterior digit of the pattern (e–h). Note an elongated metatarsal I is derived from the polarizing region (black arrow,e). (h) Digit progenitors (black numbers) adjacent to the polarizing region (green oval) transiently specified and promoted through a series of anterior identities by a gradient of paracrine Shh signalling (blue) over 12 h; in parallel, polarizing region digit progenitors (green numbers) specified and promoted through a series of anterior identities by autocrine Shh signalling over 16 h. Scale bars:a,c,g—1 mm;b—50 μm (d—same scale);e—250 μm;f—500 μm. Figure 4: Chick leg polarizing region fate maps and timing of digit specification. ( a ) Gfp -expressing polarizing regions grafted in place of host (pos, posterior) polarizing regions give rise to digit IV ( n =7/9). ( b ) Longitudinal section in situ showing Gfp expression in soft tissue and cartilage of digit IV, but not digit III ( n =2/2). ( c ) Gfp -expressing polarizing regions grafted to anterior (ant) margins give rise to duplicate (*) chick wing digit IV ( n =9/9). ( d ) Longitudinal section in situ showing Gfp expression in soft tissue and cartilage of duplicate (*) digit IV, but not duplicate digit III ( n =1/1). ( e – g ) Inhibition of Shh signalling in the leg bud using cyclopamine at stage 18/19 results in a I–I digit pattern ( e , n =2/2 and red numbers, h ), at stage 19/20, a I–II–II pattern ( f , n =4/4 and red numbers, h ) and at stage 21, a I–II–III–III pattern ( g , n =6/7 and red numbers, h ), leg polarizing region cells always give rise to the most-posterior digit of the pattern ( e – h ). Note an elongated metatarsal I is derived from the polarizing region (black arrow, e ). ( h ) Digit progenitors (black numbers) adjacent to the polarizing region (green oval) transiently specified and promoted through a series of anterior identities by a gradient of paracrine Shh signalling (blue) over 12 h; in parallel, polarizing region digit progenitors (green numbers) specified and promoted through a series of anterior identities by autocrine Shh signalling over 16 h. Scale bars: a , c , g —1 mm; b —50 μm ( d —same scale); e —250 μm; f —500 μm. Full size image Timing of chick leg digit specification by Shh signalling To examine the timing of digit IV specification in the chick leg, we replaced stage 18/19 polarizing regions with Gfp -expressing polarizing regions and added cyclopamine at a series of later time points. Cyclopamine application at stage 18/19 ( ∼ 4 h of Shh transcription) resulted in legs with a I–I digit pattern ( Fig. 4e ); at stage 19/20 ( ∼ 8 h of Shh transcription), a I–II–II pattern ( Fig. 4f ); at stage 21 ( ∼ 12 h of Shh transcription), a I–II–III–III pattern ( Fig. 4g ) and after stage 22 ( ∼ 16 h of Shh transcription), a I–II–III–IV pattern as in normal legs ( Fig. 4a ). However, we extended a previous study [18] by revealing how these digit patterns are generated by fate mapping the leg polarizing region following cyclopamine treatment. Unexpectedly, we found that, although posterior digit identities were lost, the polarizing region always gave rise to the most-posterior digit of the pattern, as in normal development ( Fig. 4a and h ): digit I at stage 18/19 ( Fig. 4e and h ), digit II at stage 19/20 ( Fig. 4f and h ) and digit III at stage 21 ( Fig. 4g,h ). The finding that the chick wing polarizing region only gives rise to soft tissues along the posterior margin of the most-posterior digit, but not the cartilage, is strong evidence that the bird wing digits are 1, 2 and 3, and not 2, 3 and 4. It is striking that the contribution the mouse forelimb polarizing region makes to digit 3 is also predominantly to soft tissues along its posterior margin [8] . Therefore, because a primary axis of cartilage condensation running through the digit 4 position is not conserved in all vertebrate limbs, the primary axis cannot be used to assign digit identity, thus eliminating the requirement of a digit frame-shift in bird wing evolution ( Fig. 1d,e ). Our results support the fossil record, indicating that birds evolved from theropod dinosaurs that lost digits 4 and 5 ( Fig. 1a ) and is consistent with the overlooked 'axis-shift' hypothesis that proposes the primary axis runs through the digit 3 position in bird wings [19] , [20] , [21] ( Figs 1f and g ). We speculate that the inability of the chick wing polarizing region to form a digit in the wing, but not in the leg, is associated with cell death that is higher along the posterior margin of the wing bud compared with the leg bud [22] . This cell death could account for the progressive decrease in the width of the stripe of cells derived from the chick wing polarizing region going from proximal to distal ( Fig. 2d ). We further speculate that this pattern of cell death evolved around 200 million years ago and eliminated posterior digits of the theropod hand/bird wing ( Fig. 1a ). We showed that three digits arise in cells adjacent to the polarizing region in both wings and legs in response to 12 h of Shh signalling ( Figs 3c and 4h ), while digit IV also arises in the polarizing region of the leg in response to 16 h of Shh signalling ( Fig. 4h ). As anterior digit identities are transiently specified at a very early stage in the chick leg polarizing region, this is likely to occur in response to short-range autocrine Shh signalling, whereas digits that arise from cells adjacent to the polarizing region arise in response to long-range paracrine Shh signalling. These processes appear parallel because blocking Shh signalling in the chick leg showed that the same digit identities are transiently specified in both the polarizing region and adjacent cells simultaneously ( Fig. 4h ). Furthermore, our findings rule out the recent suggestion that the digit 3 identity can only be specified in cells adjacent to the polarizing region in response to paracrine Shh signalling [9] . In a recent model of mouse digit patterning, it was suggested that Shh specifies all digits at a very early stage, presumably in a stepwise anterior to posterior sequence, and then is required for the survival of digit progenitor cells in the order obtained when Shh is inactivated at different time points ( Fig. 5a ) [23] . Thus, removing Shh function at progressively later stages resulted in digit patterns 1–4 then 1–2–4, with digit 4 being identified by handplate position and by genetic markers [23] , [24] ( Fig. 5a ). However, others have questioned these methods of digit identification and suggest that the digit identified as digit 4 by Zhu et al . is a more-anterior digit despite its posterior position [25] , and this would fit with earlier mouse studies ( Fig. 5b ) [8] , [18] . Indeed, our data on removing Shh function in the chick leg show that anterior digits can indeed arise from a posterior position in the polarizing region. Although our promotion model could be applied to the patterning of digits 1 to 4 of the mouse limb ( Fig. 5c ; as digits 2, 3 and 4 are indistinguishable), digit 5 has a distinct morphology and does not require the longest exposure to Shh to form [23] . Parallels have been drawn between specification of digit 5 and the neural tube floor plate [26] ; the progenitor cells in both cases experience the highest levels of Shh, but downregulate Shh target genes Gli1 and Ptc1 at an early stage [26] , [27] . Thus digit 5 progenitors, like floor plate progenitors, may be specified by a transient peak of Shh [26] , and this could occur during the time that digits 1 to 4 are being specified by promotion, both outside and inside the polarizing region ( Fig. 5d ). 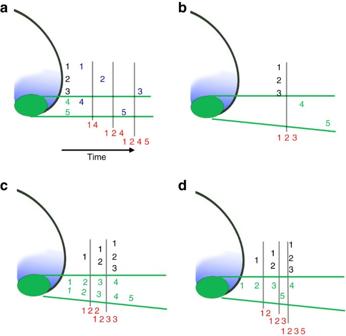Figure 5: Models of mouse limb digit patterning. (a) Biphasic model. Digit progenitors specified (black and green numbers) by a pulse of Shh signalling (blue shading) from the polarizing region (green oval). Continued Shh signalling required for specified digit progenitor cells to proliferate into cartilage condensations in the order digits 4, 2, 5 and 3 (blue numbers). Progressive removal of Shh function gives limbs with two digits, 1–4; then three digits, 1–2–4; and finally with four digits, 1–2–4–5 (red numbers). (b) Temporal expansion model. Digit progenitors 1, 2 and 3 specified by a gradient of paracrine Shh signalling adjacent to polarizing region. Digit 4 and 5 progenitors specified according to the length of time the progenitor cells are exposed to autocrine Shh signalling in the polarizing region lineage. Removal of Shh function gives limbs with three digits, 1–2–3 (red numbers, compare with 1–2–4 digit pattern ina). (c) Promotion model. Digit progenitors 1, 2 and 3 transiently specified and promoted through a series of anterior identities by concentration gradient of paracrine Shh signalling adjacent to polarizing region. In parallel, digit 4 and 5 progenitors also transiently specified and promoted through a series of anterior identities by autocrine Shh signalling in the polarizing region. Progressive removal of Shh function gives limbs with three digits, 1–2–2; and then four digits, 1–2–3–3 (red numbers). Note that digit 5 requires the longest exposure to Shh signalling. (d) Promotion and transient specification model. Same as (c), except digit 5 is specified by a transient pulse of high-level Shh signalling. Progressive removal of Shh function gives limbs with two digits, 1–2; then with three digits, 1–2–3; and finally with four digits, 1–2–3–5 (red numbers). Figure 5: Models of mouse limb digit patterning. ( a ) Biphasic model. Digit progenitors specified (black and green numbers) by a pulse of Shh signalling (blue shading) from the polarizing region (green oval). Continued Shh signalling required for specified digit progenitor cells to proliferate into cartilage condensations in the order digits 4, 2, 5 and 3 (blue numbers). Progressive removal of Shh function gives limbs with two digits, 1–4; then three digits, 1–2–4; and finally with four digits, 1–2–4–5 (red numbers). ( b ) Temporal expansion model. Digit progenitors 1, 2 and 3 specified by a gradient of paracrine Shh signalling adjacent to polarizing region. Digit 4 and 5 progenitors specified according to the length of time the progenitor cells are exposed to autocrine Shh signalling in the polarizing region lineage. Removal of Shh function gives limbs with three digits, 1–2–3 (red numbers, compare with 1–2–4 digit pattern in a ). ( c ) Promotion model. Digit progenitors 1, 2 and 3 transiently specified and promoted through a series of anterior identities by concentration gradient of paracrine Shh signalling adjacent to polarizing region. In parallel, digit 4 and 5 progenitors also transiently specified and promoted through a series of anterior identities by autocrine Shh signalling in the polarizing region. Progressive removal of Shh function gives limbs with three digits, 1–2–2; and then four digits, 1–2–3–3 (red numbers). Note that digit 5 requires the longest exposure to Shh signalling. ( d ) Promotion and transient specification model. Same as ( c ), except digit 5 is specified by a transient pulse of high-level Shh signalling. Progressive removal of Shh function gives limbs with two digits, 1–2; then with three digits, 1–2–3; and finally with four digits, 1–2–3–5 (red numbers). Full size image Our findings lead us to suggest that the digit 4 position in all vertebrate limbs is within the polarizing region, and this may be because three is the maximum number of different digits that can be specified by a concentration gradient of paracrine Shh signalling. This implies that additional digit types will always be derived from the polarizing region and specified by autocrine Shh signalling. Polarizing region grafts Fertilized transgenic Gfp -expressing chicken eggs and normal chicken eggs were incubated at 38°C, windowed and staged according to Hamburger and Hamilton [28] . GFP embryos were dissected in DMEM (Gibco) and wing and leg polarizing regions removed using fine tungsten needles, grafted to the appropriated location of stage-matched host limb buds and held in place with 25 μm platinum pins. Shh and growth inhibition At different times after polarizing region grafts were made, Shh signalling was inhibited with cyclopamine (Sigma) and growth with TSA (Sigma). TSA was dissolved in DMSO (Sigma) to make a concentration of 1 μg μl −1 . AG1-X2-beads (Sigma) were soaked in TSA for 30 min, washed twice in DMEM and then implanted into wing buds using fine tungsten needles. Cyclopamine (Sigma) dissolved in control carrier (45% 2-hydropropyl-β-cyclodextrin in PBS, Sigma) and 5 μl of a 1 μg −1 solution was pipetted directly onto embryos after removal of vitelline membranes. Alcian blue skeletal preparations Embryos were fixed in 90% ethanol for 2 days and then transferred to 0.1% Alcian blue in 80% ethanol/20% acetic acid for 1 day, before being cleared in 1% KOH. Whole-mount in situ hybridization Embryos were dissected, or wings transversely sectioned with a razor blade and fixed overnight in 4% paraformaldehyde at 4 °C. Embryos were dehydrated and rehydrated through a methanol series, washed in PBS, then treated with proteinase K for 20 min (10 μg ml −1 ) washed in PBS, fixed for 30 min in 4% PFA and then prehybridized at 65 °C for 2 h (50% formamide/50% 2× SSC). One μg of antisense mRNA probes for Shh and Gfp were added to 1 ml of hybridization buffer (50% formamide/50% 2× SSC) at 65 °C overnight. Embryos were washed in hybridization buffer (minus mRNA probes) and then in maleic acid buffer (MAB) buffer, before being transferred to blocking buffer (2% blocking reagent, 20% lamb serum in MAB buffer) for 2 h at room temperature. Embryos were transferred to blocking buffer containing anti-digoxigenin antibody (1/2,000) at 4 °C overnight, then washed in MAB buffer before being transferred to NTM (NaCl, Tris, MgCl 2 ) buffer containing nitro-blue tetrazolium/5-bromo-4-chloro-3-indolyl phosphate and mRNA distribution visualized. Section in situ hybridization Dissected limbs were embedded in paraffin wax, and 14 μm longitudinal sections were cut and mounted onto aminoalkylsilane-coated slides and de-waxed at 60 °C. Slides were washed in Histoclear, rehydrated through an ethanol series and then washed in PBS. Slides were treated with proteinase K (10 μg ml −1 ), and whole-mount protocol followed thereon. How to cite this article: Towers, M. et al . Insights into bird wing evolution and digit specification from polarizing region fate maps. Nat. Commun. 2:426 doi: 10.1038/ncomms1437 (2011).